Localization and topology protected quantum coherence at the edge of hot matter Topological phases are characterized by edge states confined near the boundaries by a bulk energy gap. On raising temperature, these edge states are typically lost due to mobile thermal excitations. However, disorder can localize an isolated many-body system, potentially allowing for a sharply defined topological phase even in a highly excited state. We explicitly demonstrate this in a model of a disordered, one-dimensional magnet with spin one-half edge excitations. Furthermore, we show that the time evolution of a simple, highly excited state reveals quantum coherent edge spins. In particular, we demonstrate the coherent revival of an edge spin over a time scale that grows exponentially with system size. This is in sharp contrast to the general expectation that quantum bits strongly coupled with a hot many-body system will rapidly lose coherence. This result opens new directions in the study of topologically protected quantum dynamics. Observing coherent quantum phenomena generally requires arranging for some degree of isolation—either physical isolation, to reduce coupling with other degrees of freedom, or by cooling to very low temperatures to freeze out excitations. Therefore, quantum coherence is not expected to survive for long in a general many-body system placed in an excited state. In particular, quantum bits embedded in such a dynamical system are expected to rapidly decohere. This follows from the assumption of ergodicity—even a closed many-body system evolving in time under the Schrödinger equation is assumed to approach thermal equilibrium independent of most details of the initial state [1] , [2] , [3] , [4] . In particular, no quantum interference is expected because the outcome would then depend on the initial preparation, in contrast to the expectation for an equilibrium state. Yet, not all many-body systems necessarily thermalize. A well-studied exception to this rule are the so-called integrable systems. But these are very specific, fine-tuned models whose special properties are lost on adding generic perturbations that are present in a real world realization. A more physically robust mechanism by which quantum coherence can avoid a thermal death is through localization. Anderson, in his original paper on quantum localization [5] , conjectured that closed many-body quantum systems with a sufficiently strong random potential will fail to thermalize. The idea was revived by Basko et al . [6] , who gave new theoretical arguments for the stability of the many-body localized (MBL) state in interacting systems decoupled from an external bath. Numerical studies have provided further support for the existence of a non-thermalizing MBL state [7] , [8] . Even if it does not thermalize, a many-body system still has incredibly complex dynamics. With a huge number of correlated degrees of freedom, it is not clear that the system can have any retrievable quantum coherence. Indeed, the time evolution of a many-body system generally involves unbounded growth of the (entanglement) entropy even in the localized state [9] , [10] , [11] , [12] , which may suggest irreversible loss of information. To measure and utilize quantum coherence will require at least one addressable degree of freedom that is effectively decoupled from all the rest. Again, this appears to require immense fine tuning. Nonetheless, here we show that a MBL state with a certain topological character can guarantee a dynamically decoupled degree of freedom at the edge, which, therefore, retains its quantum coherence. This is a result of having topological properties that persist to arbitrarily high-energy eigenstates. In the more familiar context of ground state topological phases, edge modes are protected by a bulk gap and the symmetries of the system [13] , [14] , [15] , [16] , [17] , [18] . An example relevant to our discussion is the antiferromagnetic spin-1 chain, which has an energy gap to bulk excitations [19] but which, remarkably, hosts a free spin-1/2 state at the edge [20] . The fractional edge spin is a manifestation of a topological property of the ground state, which survives as long as certain discrete spin rotation symmetries are present. Hence, this defines a symmetry protected topological (SPT) phase. However, in a clean system at any finite temperature, the edge spins mix with delocalized bulk states, and no sharp definition of this phase remains. In the model system we present below, a similar edge spin-1/2 quantum bit appears, but it is preserved even on heating the bulk due to localization of the bulk modes. Here in the absence of thermal equilibrium, the analogue of a high-temperature state is one with an energy that significantly exceeds the ground state, so that even in the thermodynamic limit a finite excitation energy density (energy per spin) remains. The existence of topological order in individual high-energy eigenstates due to many-body localization was also recently proposed in refs 21 , 22 , where certain characteristic properties of such localized topological eigenstates were discussed. It is, however, important to emphasize that preparing a many-body system in an energy eigenstate, while possible in small size numerical simulations, is experimentally an impossible task because it would require to perform highly non-local operations on the system. Thus, while a distinction between phases may appear in correlations measured in individual eigenstates as outlined in refs 21 , 22 , they leave open the question of a physical distinction between them that can be probed in an experiment working with a generic initial state. Here we identify just such a dynamical property that also serves as a smoking gun signature of the topological phase. In particular, the coherence of the edge spin and its robustness to generic interactions in the system is clearly demonstrated below using theoretical arguments and confirmed by numerical simulation of the quantum dynamics using exact diagonalization of a spin chain with quenched disorder. Irreversible decoherence occurs only after a time exponentially long in the system size, indicating that the edge degree of freedom can maintain perfect coherence in the infinite system limit. Model To demonstrate the existence of edge states at high-energy densities and to show how they can be manipulated coherently, we shall work with the following spin chain Hamiltonian Here represent Pauli matrices at site i of a one-dimensional chain and the parameters λ i , h i and V i are independent random variables. Note, there are two Z 2 symmetries corresponding to independently on the even- and odd-numbered sites. We note that the first two terms of (1) can be mapped to a non-interacting (Majorana) fermion model using a Jordan–Wigner transformation [23] . (We remark, however, that probe fields coupling with the edge states in the spin variables may appear in an unnatural, non-local manner in the fermionic variables, which limits the usefulness of the mapping.) The last term V i adds interactions between the fermions, making the model generic. The arguments of Basko et al . [6] for the stability of many-body localization apply here, as we will work in the limit of weak interactions and strong disorder. There are two simple limits in which the Hamiltonian (1) can be trivially diagonalized, which represent two distinct dynamical phases. First, if the only terms in (1) are the local fields h i , then the system is in a trivial localized state. All eigenstates are then simple product states of the spins in the σ x basis. The other limit, in which only the three-spin terms λ i are non-zero, represents a non-trivial localized phase protected by Z 2 × Z 2 symmetry, analogous to the Haldane phase of the spin-1 chain. In this phase, all the eigenstates are cluster states with distinct topological properties that are manifested by the presence of edge states. Crucially, the distinction between the two types of spectra can persist away from the simple limit and in the presence of interactions V i due to the localized nature of the state. Such protection of quantum order by many-body localization was discussed in refs 21 , 22 . 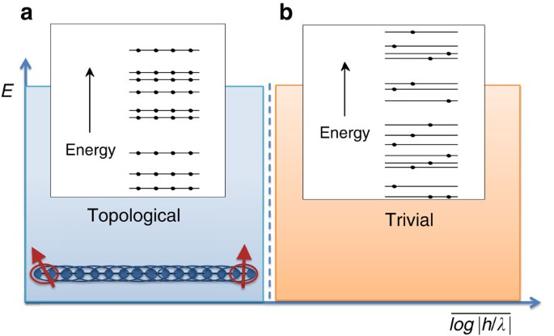Figure 1: Schematic phase diagram of the model in equation 1. Vertical axis is energy density such that the maximum corresponds to infinite temperature in an equilibrium system. Horizontal axis is a measure of the typical strength of the transverse field to the three-spin term. With strong disorder, all eigenstates are localized but change character from the left to right end. In contrast to the trivial phase (b), the topological phase (a) is characterized by quadrupling of energy levels (horizontal lines) sufficiently deep in this phase. Solid dots are used to highlight the levels and the degeneracy; they are displaced along the horizontal direction for visibility. Spectrum is shown close toE=0 in model equation 1, with parameter s.d.σV=0.1 and (σλ,σh)=(1.0, 0.05) on the left and (0.1, 1.0) on the right. Figure 1 gives a schematic view of the phase diagram showing the transition from the trivial to the topological eigenstates of the model (1) with decreasing transverse field h i . The transition between the two localized phases can occur through a direct transition described by an infinite randomness dynamical critical point [24] , [25] , while an intervening delocalized phase appears unlikely [21] . In the sections below, we describe the non-trivial dynamics that ensues when the system is in the topological phase, stressing, in particular, the behaviour of the protected edge modes. Figure 1: Schematic phase diagram of the model in equation 1. Vertical axis is energy density such that the maximum corresponds to infinite temperature in an equilibrium system. Horizontal axis is a measure of the typical strength of the transverse field to the three-spin term. With strong disorder, all eigenstates are localized but change character from the left to right end. In contrast to the trivial phase ( b ), the topological phase ( a ) is characterized by quadrupling of energy levels (horizontal lines) sufficiently deep in this phase. Solid dots are used to highlight the levels and the degeneracy; they are displaced along the horizontal direction for visibility. Spectrum is shown close to E =0 in model equation 1, with parameter s.d. σ V =0.1 and ( σ λ , σ h )=(1.0, 0.05) on the left and (0.1, 1.0) on the right. Full size image We stress that the properties that we demonstrate are more universal than our choice of model. Our theoretical arguments rely only on symmetry and the general characterization of MBL systems without a many-body mobility edge via a complete set of quasi-local integrals of motion [11] , [26] , [27] . The dominant three-spin interactions in our model are by no means a fundamental requirement for establishing the strongly disordered topological phase but rather offer a convenient theoretical starting point with vanishing correlation length. These terms are likely to be continuously connected to a more natural but finite correlation length model. Idealized cluster limit To understand the dynamics in the Hamiltonian (1) and the nature of the eigenstates, consider first the simplified version having only the first term of (1), that is, H 0 =∑ i λ i K i , where are mutually commuting operators called stabilizers. Since this model is a sum of stabilizers, the eigenstates are mutual eigenstates of all the K i ’s labelled by the respective eigenvalues ±1. These states are called cluster states in the quantum information literature. Cluster states have non-trivial entanglement properties since the K i are spatially overlapping. In fact, they are an example of SPT states [13] , [14] , [15] with Z 2 × Z 2 symmetry [28] . The topological nature of the cluster states is encapsulated in a string-order parameter [29] given by , assuming the symmetry remains unbroken. In a specific eigenstate and disorder realization, the string-order parameter takes random values O st ( i , j )=±1. Hence, we can form the non-local analogue of the Edwards–Anderson glass-order parameter , which gains a non-zero expectation value in the topological glass. This order is found in eigenstates of H 0 at all energies. Another manifestation of topological order that can be seen is in the entanglement spectrum [30] . If we pick an eigenstate of the system with periodic boundary conditions, for instance, and consider the reduced density matrix obtained by tracing over half of the system, the resulting entanglement spectrum (eigenvalues of the density matrix) will be fourfold degenerate in the topological phase due to the spin one-half at each end of the cut (see Supplementary Fig. 1 ). The non-trivial structure of the cluster states gives rise to edge modes that behave as free spin-1/2 particles. This is easily seen by constructing a spin-1/2 algebra of edge operators: on the left edge and similarly on the right edge. We say that these edge degrees of freedom behave as free spins because H 0 commutes with them. Note that the Σ L operators cannot individually appear in the Hamiltonian since they break the underlying Z 2 × Z 2 symmetry. As an example of the dynamics in this model, we can consider the time evolution starting from an initial product state with the first spin polarized along x and all the rest polarized along z . In this state, the left edge q-bit is oriented along and will remain in this state independent of the complicated dynamics of the bulk spins. Effect of interactions We now consider adding to the Hamiltonian H 0 generic perturbations such as h i and V i in (1), which destroy its integrability but preserve the Z 2 × Z 2 symmetry of the problem. An important simplification occurs in the limit of strong disorder (relevant to the models discussed here), when eigenstates at all energies are localized. Then, one can identify integrals of motion in a MBL state [11] , [26] , [27] that take on a quasi-local character. This will provide a powerful conceptual tool to also describe the localized topological phase and interpret numerical results for the dynamics. The eigenstates of the toy model discussed above were the strictly localized cluster states. Assuming localization persists on adding the interaction terms, the local stabilizers K i will map to a set of commuting integrals of motion that are still local up to an exponentially decaying tail. Like the original stabilizers K i , each is one projection of a spin-1/2 variable. We term such operators quasi-local. Similarly, we will have modified quasi-local left edge operators that remain decoupled from the dynamical (bulk) Hilbert space in a semi-infinite system. Because the topological structure of the eigenstates is unchanged by the interactions, the entanglement spectra must retain the fourfold degeneracy (see Supplementary Fig. 1 ). Experiments can have direct access only to simple, strictly local operators such as the original edge operators and not to the exact decoupled operators . The crucial point is that if the system is in the localized phase, the measurable quantity has an overlap with the true edge operator. That is, we can write the original edge operator as a sum of a left edge contribution and a bulk contribution . If we start the dynamics with fully polarized in the α direction, then a polarization of Z α will remain after arbitrarily long-time evolution. If, on the other hand, the system is finite, the non-local tails of the new edge operators can lead to interactions between the two edges and the bulk of the system through terms of the form A large number of non-local bulk operators B m are possible and the respective coefficients are all exponentially small in the system size. The different terms give rise to oscillations at a large number of frequencies, which will in turn lead to decay of the edge spin over a time τ N that scales exponentially in the system size N . For the integrable system with V i =0, only a few interedge coupling terms can occur. This is observed explicitly in the oscillation of the edge spin at a small number of frequencies (see Supplementary Fig. 2 ). Results from numerical diagonalization of the model (1) with up to 11 spins are shown in Fig. 2 . In one set of calculations, done in a parameter regime deep in the topological phase, the system is initialized in a product state with all spins polarized along σ z , so that the bare edge operator has a definite value +1. In another set of calculations, we retain the initial conditions above except for the first spin, which is polarized along σ x so that has a definite value. In both cases, the spin expectation value first drops to a smaller non-vanishing value, which later decays to zero on a much longer time scale, which we label T 0 ( Fig. 2a ). ( Supplementary Fig. 3 shows how T 0 was extracted from the numerical results). Analysis of T 0 as a function of system size confirms the exponential size dependence discussed above. In contrast, the spin expectation value in the bulk of the system always decays rapidly to zero. In the trivial phase ( larger than a critical value), a uniform initial polarization of σ z decays both in the bulk and at the edge ( Supplementary Fig. 4 ). Note that while may persist in the trivial phase, both in the bulk and on the edge, other spin components are not conserved and hence there is no preserved quantum spin. 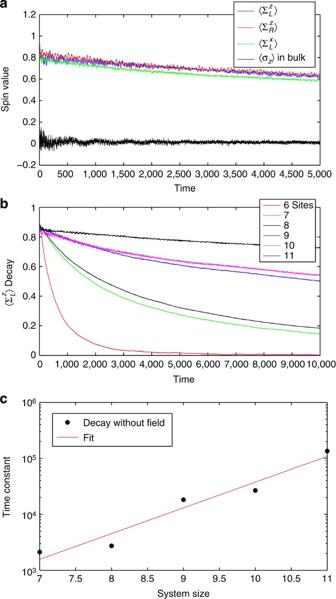Figure 2: Decay of a quantum edge spin in the topological phase. (a) Disorder averagedσzat the ends (labelled) and near the centre of the ten-site chain show the rapid decay of spin in the bulk but long-lived edge spins for an initial state with all spins polarized alongz. For a different initial state,will persist instead, as shown, demonstrating the quantum nature of the edge spin. (Drop from initial +1 value not visible on this time axis scale). (b) The disorder averaged edge spin decay for different system sizesL(c) shows an exponential dependence of the time constantT0(L) on system size, which is independent of an apparent even–odd effect, indicating that the long-time decay of the edge spin originates from coupling with the opposite edge spin via the bulk. Parameters used had zero mean and s.d. were (σλ,σV,σh)=(1.0, 0.1, 0.05). Figure 2: Decay of a quantum edge spin in the topological phase. ( a ) Disorder averaged σ z at the ends (labelled ) and near the centre of the ten-site chain show the rapid decay of spin in the bulk but long-lived edge spins for an initial state with all spins polarized along z . For a different initial state, will persist instead, as shown, demonstrating the quantum nature of the edge spin. (Drop from initial +1 value not visible on this time axis scale). ( b ) The disorder averaged edge spin decay for different system sizes L ( c ) shows an exponential dependence of the time constant T 0 ( L ) on system size, which is independent of an apparent even–odd effect, indicating that the long-time decay of the edge spin originates from coupling with the opposite edge spin via the bulk. Parameters used had zero mean and s.d. were ( σ λ , σ V , σ h )=(1.0, 0.1, 0.05). Full size image Quantum coherent dynamics and spin echo The fact that all components of the topological edge states are conserved in the dynamics suggests that this degree of freedom can indeed store a quantum bit of information. Can it also be manipulated coherently as a q-bit? To answer this question, consider coupling the addressable edge spin to a local field . Since we are in the MBL phase, there is still a constant of motion directly related to . But because the field breaks the protecting Z 2 × Z 2 symmetry, it induces coupling between the edge operator and the bulk Now, instead of observing oscillations at a single frequency ω = g as in the idealized cluster model, the edge spin should precess with many frequencies, leading to decoherence. The decoherence time is independent of system size, set only by the magnitude of the field g and the intrinsic interactions that determine the coefficients . At a glance, such dephasing with an infinite number of intrinsic modes appears deadly to the quantum coherence of the q-bit. However, note that all the terms causing the dephasing of the edge modes are proportional to the external field g , or more generally to an odd power of it (see Supplementary Note 1 ). Hence, by reversing that field, all oscillations terms are reversed, leading to a spin echo. The overlap between initial and final spins is less than unity but finite and expected to persist to infinite time in the thermodynamic limit. In a finite-size system, there is an additional imperfection due to the field-independent coupling between the two edges, which is exponentially small in the system size. Note that this echo protocol relies on the fact that in the absence of the external edge field, which breaks the protecting symmetry, the q-bit behaves as a completely free spin. The standard spin-echo protocol in contrast would produce an echo regardless of whether the edge spin were topological and would also give an echo of bulk degrees of freedom [31] . Hence, the protocol we propose serves as another sensitive diagnostic of the topological origin of the edge state. To numerically test the degree of edge coherence, we computed the time evolution of the edge spin in the model (1) supplemented by a local field applied at one end of a chain. 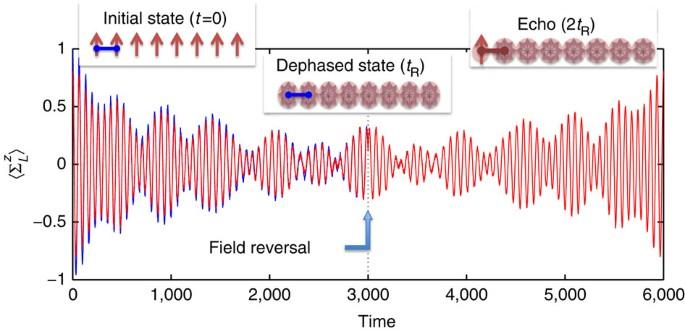Figure 3: Hidden quantum coherence. The system is prepared with all spins polarized alongz. Hence, the initial expectation value of the edge spin. The state is evolved with the Hamiltonian in the topological phase and an edge field along. The edge spin precesses and decays with a length independent time constant. However, reversing the edge fieldg→−gat timet=tRleads to a spin echo at timet=2tR, which recovers much of the lost amplitude. The oscillations of the edge spinare shown here for a particular disorder realization before (blue) and after (red) the field reversal. The red trace is reflected about the time axis to show retracing of the edge spin in the dynamics. Figure 3 shows an example of the dynamics in a specific disorder realization for an eight-site chain, starting from a definite value of the left edge . As expected, we see oscillations of decaying on a time scale that is independent of the system size (see Supplementary Fig. 5 ). This is a dephasing time in NMR terminology. At time t R , we reverse the field g and observe a near-perfect retracing of the oscillations. The edge spin echo at 2 t R degrades slowly with increasing the reversal time t R , from which we can extract a relaxation time, called T 2 by analogy with NMR terminology (see Supplementary Fig. 6 ). It is remarkable that here T 2 increases exponentially with growing system size, as shown in Fig. 4 . This implies that in the large size limit, the edge q-bit can maintain truly perfect coherence in spite of it being embedded in an interacting many-body system with high-energy density. Figure 3: Hidden quantum coherence. The system is prepared with all spins polarized along z . Hence, the initial expectation value of the edge spin . The state is evolved with the Hamiltonian in the topological phase and an edge field along . The edge spin precesses and decays with a length independent time constant . However, reversing the edge field g →− g at time t = t R leads to a spin echo at time t =2 t R , which recovers much of the lost amplitude. The oscillations of the edge spin are shown here for a particular disorder realization before (blue) and after (red) the field reversal. The red trace is reflected about the time axis to show retracing of the edge spin in the dynamics. 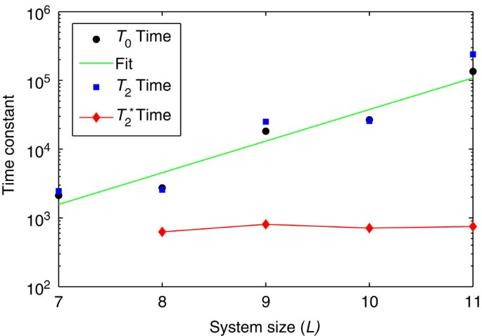Figure 4: Scaling of all the time constants with system size. The zero-field decay timeT0and spin-echo decay timeT2are nearly identical and scale exponentially with system size, whereas the oscillations decay timeis size independent. Parameters used had zero mean and s.d. were (σλ,σV,σh)=(1.0,0.1,0.05). Full size image Figure 4: Scaling of all the time constants with system size. The zero-field decay time T 0 and spin-echo decay time T 2 are nearly identical and scale exponentially with system size, whereas the oscillations decay time is size independent. Parameters used had zero mean and s.d. were ( σ λ , σ V , σ h )=(1.0,0.1,0.05). Full size image It is interesting to note that in spite of the numerous integrals of motion the bulk of the system reaches, for all practical purposes, an infinite temperature. This is because the initial product states we prescribed do not constrain the value of those integrals of motion. The edge q-bit on the other hand remains ‘cold’ due to the dynamical decoupling from the bulk. Unlike in a trivial MBL phase where a spin-echo protocol would be required even to recover quantum memory stored in the bulk degrees of freedom, here it is needed only to undo decoherence induced by the field used to manipulate the q-bit and which breaks the protecting symmetry. The presence of the underlying topological phase is crucial for providing a (edge) quantum bit that can be manipulated. We have shown that a topological edge state can survive as a coherent degree of freedom at arbitrarily high energies due to localization of the bulk modes. Our results are far more general than the specific model because our numerical demonstration is supported by theoretical analysis relying only on two powerful concepts, namely (i) symmetry and (ii) the existence of a complete set of quasi-local integrals of motion in the MBL state. These arguments together with the numerical results show that the topological phase we identify is not fine tuned. There is a finite region of parameter space in which the existence of high-energy topological edge states and high-energy quantum coherence will be realized. By extending the notion of topological edge states from gapped ground states to the full many-body spectrum, our results open the way to investigations of topological effects in dynamics. Remarkably, these unusual dynamical signatures are visible even in the absence of cooling, as long as the system of interest is described by a spin Hamiltonian in this phase. This may have practical consequences in terms of their experimental realizability, for example, in ultracold atomic gases, where cooling below the scale of magnetic interactions poses technical challenges. At the same time, systems of ultracold atoms or ions quite naturally fulfill the requirement of being decoupled from an external bath. A literal realization of model (1) with trapped ions can utilize techniques demonstrated in ref. 32 . Finally, the topological states of the spin chain (1) are related to a much wider classification of SPT ground states [13] , [14] , [15] , [16] , [17] , [18] . An interesting question for future investigation is whether the interplay of localization and topology in the higher dimensional members of this classification [33] , [34] , [35] , [36] , [37] , [38] can help protect the edge states from mixing with the bulk and thereby lead to novel dynamical phenomena at high-energy densities. How to cite this article: Bahri, Y. et al . Localization and topology protected quantum coherence at the edge of hot matter. Nat. Commun . 6:7341 doi: 10.1038/ncomms8341 (2015).